Enhanced carrier multiplication in engineered quasi-type-II quantum dots One process limiting the performance of solar cells is rapid cooling (thermalization) of hot carriers generated by higher-energy solar photons. In principle, the thermalization losses can be reduced by converting the kinetic energy of energetic carriers into additional electron-hole pairs via carrier multiplication (CM). While being inefficient in bulk semiconductors this process is enhanced in quantum dots, although not sufficiently high to considerably boost the power output of practical devices. Here we demonstrate that thick-shell PbSe/CdSe nanostructures can show almost a fourfold increase in the CM yield over conventional PbSe quantum dots, accompanied by a considerable reduction of the CM threshold. These structures enhance a valence-band CM channel due to effective capture of energetic holes into long-lived shell-localized states. The attainment of the regime of slowed cooling responsible for CM enhancement is indicated by the development of shell-related emission in the visible observed simultaneously with infrared emission from the core. A fundamental source of limited efficiency in solar cells is their transparency towards solar radiation on the redder side of the solar spectrum, specifically for photon energies ( ħω ) below the band gap ( E g ) of the active absorbing material ( Fig. 1a ) [1] . Methods such as stacking semiconductors with different energy gaps within a photovoltaic device (that is, tandem cells) [2] , [3] or the incorporation of a partially filled band within the energy gap of the absorbing material (so-called intermediate-band cells) [4] , [5] have been explored for improved harvesting of these lower-energy solar photons. Another major source of energy loss is associated with the rapid cooling, or thermalization, of hot charge carriers generated by photons with energies well above E g ( Fig. 1a ). Concepts for mitigating thermalization losses involve either hot-electron extraction for increasing photovoltage (in hot-carrier devices) [6] , [7] or use of impact ionization to increase photocurrent [8] , [9] , [10] , [11] . In the latter process, Coulombic collisions of hot photoexcited carriers with electrons within the valence band excite them across the energy gap, generating additional electron-hole pairs ( Fig. 1b ). This results in increased photocurrent that can potentially boost the power conversion limit of solar cells from ca . 30% (ref. 1 ) to >40% (refs 8 , 12 ). The interest in this phenomenon, termed carrier multiplication (CM) or multiexciton generation, has been stimulated by recent advances in the understanding of the photophysics of nanostructures that demonstrate how CM can benefit from the effects of quantum confinement. As first suggested by Nozik [9] , one advantageous factor is the reduced rate of carrier cooling due to inhibition of phonon emission, which becomes less efficient as the separation between electronic states widens. Other factors include relaxation of momentum conservation [13] and reduced dielectric screening [14] , both of which should increase the rate of impact ionization and, hence, CM efficiency. 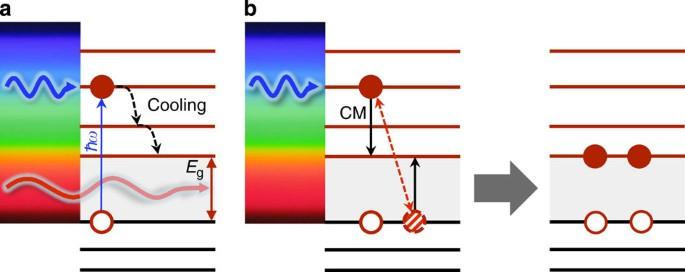Figure 1: Photon-to-charge-carrier conversion without and with carrier multiplication. (a) Energy losses in a photovoltaic device arise from fast cooling of hot carriers generated by high-energy photons withħω>Eg(thermalization loss) and the fact that low-energy photons withħω<Egare transmitted through the active layer without being absorbed (transparency loss). (b) CM can be explained in terms of an impact-ionization-like scattering between a hot carrier (a conduction-band electron in the example in the figure) and a pre-existing valence band electron, which is promoted to the conduction band producing an additional electron-hole pair. Figure 1: Photon-to-charge-carrier conversion without and with carrier multiplication. ( a ) Energy losses in a photovoltaic device arise from fast cooling of hot carriers generated by high-energy photons with ħω > E g (thermalization loss) and the fact that low-energy photons with ħω < E g are transmitted through the active layer without being absorbed (transparency loss). ( b ) CM can be explained in terms of an impact-ionization-like scattering between a hot carrier (a conduction-band electron in the example in the figure) and a pre-existing valence band electron, which is promoted to the conduction band producing an additional electron-hole pair. Full size image Indeed, as was indicated by the first measurements of zero-dimensional PbSe quantum dots (QDs) [15] in 2004 and follow-up QD studies [16] , [17] , [18] , [19] , [20] , [21] , [22] , [23] , nanomaterials can show CM efficiencies that surpass those of bulk solids. A key development in reaching this important conclusion was the elucidation of the role of uncontrolled photocharging of QDs [24] , [25] , which was a major source of discrepancies in earlier CM measurements [17] , [26] , [27] , [28] , [29] , [30] if its effects were not ameliorated by using stirred [24] , [25] , [26] , [27] , [31] or flowed [32] QD solution samples. Enhanced CM efficiencies have also been observed in several other types of nanostructures, including quasi-one-dimensional (1D) nanorods [33] , [34] , 1D carbon nanotubes [35] , and two-dimensional graphene [36] . Recent studies of QD-based photodetectors [11] as well as sensitized-titania [37] and p–n junction [10] solar cells have shown that CM can produce greater-than-unity quantum efficiencies in photon-to-charge-carrier conversion, firmly establishing its relevance to practical photovoltaic technologies. An outstanding challenge in the CM field is the development of nanomaterials that show high CM efficiencies within the range of photon energies relevant to solar energy conversion ( ħω <4 eV). The CM performance can be quantitatively characterized in terms of an energetic threshold ( ħω th ) and an electron-hole pair creation energy ( ε eh ). The latter is defined as the energy in excess of ħω th required to generate a new carrier pair, and it can be derived from the inverse slope of the dependence of quantum efficiency of photon-to-exciton conversion ( q ) plotted versus ħω : ε eh =( dq / dħω ) −1 . The values of ε eh and ħω th are interconnected, and typically a reduction in ε eh translates into a reduced CM threshold [38] . On the basis of energy conservation, the minimal values of ε eh and ħω th are E g and 2 E g , respectively. These fundamental limits are the current targets in the development of new highly efficient CM materials. Here we demonstrate that the use of wavefunction engineering in core/shell QDs represents a promising approach to reaching these targets. Core/shell approach to CM engineering A recently proposed phenomenological window-of-opportunity model [39] relates ε eh to the non-CM (for example, phonon-related) energy-loss rate ( k cool ; measured, e.g., in units of eV/ps) and the CM rate ( r CM =1/ τ CM ; τ CM is the characteristic CM time) by an intuitive expression ε eh = k cool/ r CM = k cool τ CM . In the case of phonon-assisted cooling, k cool = ħω 0 / τ 0 , where ħω 0 and τ 0 are the phonon energy and the phonon emission time, respectively [40] . This model suggests that one can reduce ε eh by either increasing the CM rate, perhaps by increasing the strength of Coulomb coupling between interacting charges, or by decreasing the rate of cooling. The importance of the cooling factor has been demonstrated by recent comparative studies of PbS, PbSe and PbTe QDs [31] , [39] , [40] , which showed that the observed difference in CM yields can be directly related to the difference in energy-loss rates. In the present work, we simultaneously manipulate k cool and r CM using appropriately designed core/shell QDs that consist of an infrared-active PbSe core overcoated with an especially thick shell of wider-gap CdSe ( Fig. 2a ). Available spectroscopic data in conjunction with electronic structure calculations suggest that the conduction band offset at the PbSe/CdSe interface is close to zero [41] , [42] . As a result, the wavefunction of the band-edge electron 1 S e state in these QDs occupies the entire volume of the core/shell structure, while the band-edge hole wavefunction (1 S h ) is closely confined to the core due to a large (~1.48 eV) valence-band offset at the core/shell interface (see Fig. 2a , where we show an approximate structure of electronic states calculated using a simple, single-band effective mass approximation). This regime of confinement, which is characterized by a partial spatial separation between the electron and hole wavefunctions, is typically referred to as quasi-type-II (ref. 43 ). 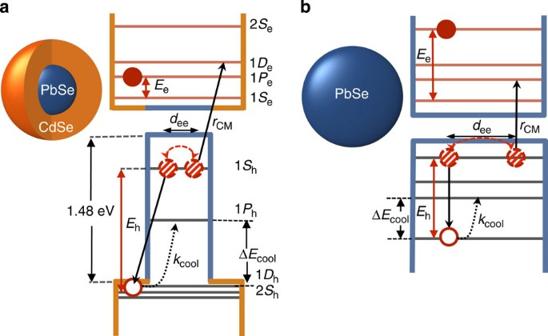Figure 2: Schematic representations of electronic states in core/shell and core-only QDs. (a) Representation of a PbSe/CdSe core/shell QD with a thick shell and the approximate structure of electronic states for a QD with 2 nm core radius and 2 nm shell thickness. The QD energy spectrum features closely spaced electron levels and sparsely distributed hole core levels (with a typical energy separation depicted as ΔEcool). Red arrows indicate excess energies for the electron and the hole,EeandEh, respectively, demonstrating the asymmetric distribution of the photon excess energy (ħω−Eg) between the two carriers (Eh>Ee), which could allow for shifting the CM threshold closer to the fundamental 2Eglimit. Relaxation of a hot hole from a shell-based state to a core-localized level can happen either via a CM process (straight black lines) or thermalization (dotted black line). Here, the pre-existing core-localized valence-band electrons interacting in the CM process are spatially separated by the distancedee, which is much smaller than the overall QD size. The photogenerated and pre-existing carriers are shown by solid and dashed circles, respectively. (b) Band structure and relaxation processes in a core-only PbSe QD of the same overall size. For this structure, the salient differences are mirror-symmetric conduction and valence-band states, which results in a symmetric distribution of the photon excess energy between the electron and the hole, and a larger spatial separation of the carriers interacting in CM. Figure 2: Schematic representations of electronic states in core/shell and core-only QDs. ( a ) Representation of a PbSe/CdSe core/shell QD with a thick shell and the approximate structure of electronic states for a QD with 2 nm core radius and 2 nm shell thickness. The QD energy spectrum features closely spaced electron levels and sparsely distributed hole core levels (with a typical energy separation depicted as Δ E cool ). Red arrows indicate excess energies for the electron and the hole, E e and E h , respectively, demonstrating the asymmetric distribution of the photon excess energy ( ħω − E g ) between the two carriers ( E h > E e ), which could allow for shifting the CM threshold closer to the fundamental 2 E g limit. Relaxation of a hot hole from a shell-based state to a core-localized level can happen either via a CM process (straight black lines) or thermalization (dotted black line). Here, the pre-existing core-localized valence-band electrons interacting in the CM process are spatially separated by the distance d ee , which is much smaller than the overall QD size. The photogenerated and pre-existing carriers are shown by solid and dashed circles, respectively. ( b ) Band structure and relaxation processes in a core-only PbSe QD of the same overall size. For this structure, the salient differences are mirror-symmetric conduction and valence-band states, which results in a symmetric distribution of the photon excess energy between the electron and the hole, and a larger spatial separation of the carriers interacting in CM. Full size image The use of quasi-type-II nanostructures can benefit CM for multiple reasons, as schematically illustrated in Fig. 2a,b via a comparison with standard PbSe QDs that are currently among the best CM performers. First, confining the ground-state hole wavefunction to a comparatively small volume increases the energetic gap between the hole states immediately below the band edge of the shell material (Δ E cool , Fig. 2a ), slowing down hole relaxation from the higher lying states due to a phonon bottleneck [44] . Moreover, reduced wavefunction overlap between the higher-lying, shell-based and lower, core-localized hole states will further slow hole relaxation. Finally, the core-localized valence band carriers involved in CM should experience increased Coulomb coupling due to decreased spatial separation between them ( d ee in Fig. 2a,b ). Another important aspect of these quasi-type-II structures is a reduced CM threshold compared with standard PbSe QDs. The mirror symmetry between the conduction and valence bands of PbSe [45] , along with optical selection rules, dictate that the energy of an absorbed photon in excess of E g will be partitioned approximately equally between an electron and a hole, that is, E e = E h =( ħω − E g )/2 ( Fig. 2b ). Since at the CM threshold either E e or E h must be at least equal to E g , it follows that ħω th is ca. 3 E g . In thick-shell PbSe/CdSe QDs, absorption at high CM-relevant energies is dominated by the CdSe shell. Therefore, excitation of one of the optically allowed transitions near the shell band edge leads to a strongly asymmetric case where E h is much greater than E e (see Fig. 2a ); as ( ħω − E g ) is no longer equally divided between E e and E h , ħω th can more closely approach the fundamental 2 E g limit. Furthermore, the large overall size of the QD results in a close energy spacing between electron and hole states of different symmetries near the CdSe band edges, which makes it much easier to simultaneously meet the requirements of both optical and Coulombic selection rules [16] , [46] . Synthesis and optical spectroscopy of PbSe/CdSe QDs The PbSe/CdSe QDs studied in this work were synthesized via a modified version of a previously reported method (see Methods) [47] . Briefly, we first fabricate large PbSe QDs with radii from 3.5 to 5 nm, and then apply partial cation exchange to create an outer CdSe shell of controlled thickness by exchanging ions of Pb 2+ with Cd 2+ . Using a moderate reaction temperature (130 °C), we can achieve a wide range of shell thicknesses while avoiding the formation of homogeneous CdSe particles. This procedure preserves the overall diameter of the QDs and allows us to gradually tune the aspect ratio of the resulting core/shell structure ( ρ ), defined as the ratio of the shell thickness ( H ) to the total radius ( R ): ρ = H/R . Both the starting PbSe QDs and the final PbSe/CdSe structures exhibit a nearly spherical shape and fairly narrow size dispersity (s.d. of the overall size is ~7%; see transmission electron microscopy (TEM) images, in Fig. 3a ). The core and shell sizes within a given sample appear less uniform, exhibiting ca. 15% dispersion. 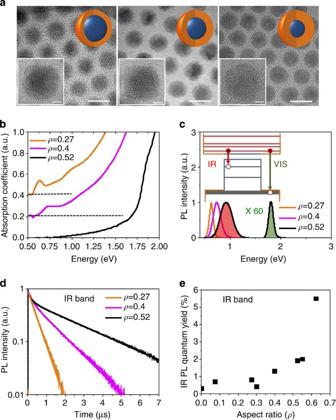Figure 3: Structural and spectroscopic characterization of core/shell QDs. (a) TEM images showing typical core/shell QDs with aspect ratios of 0.27, 0.4 and 0.52, and a constant overall radius of 4 nm. Scale bars, 10 nm. Insets are higher resolution images (scale bars, 2 nm) of individual QDs. (b) Absorption spectra for the same QDs, indicating a blue shift and a decrease in amplitude of the first excitonic peak associated with the 1Se−1Shtransition with increasing shell thickness. Spectra are shifted vertically for clarity. (c) PL spectra for the same QDs, showing progressive blue shifts with increasing shell size and the emergence of visible emission for the QDs with the thickest shell (shaded spectra). Inset shows a schematic representation of the band structure, indicating the transitions associated with the infrared and visible emission. All infrared spectra are normalized, whereas for the thick-shell structure the visible emission amplitude is multiplied by a factor of 60 for the purpose of comparison. (d) Infrared PL traces (core emission) are characterized by microsecond time constants and indicate a progressive increase in single-exciton lifetime (from 0.42 to 1.2 μs, and then 2.6 μs for the plotted traces) for structures with larger shell thicknesses, which is a typical signature of a quasi-type-II regime. (e) The PL quantum yield of the infrared band increases with increasing aspect ratio. Figure 3: Structural and spectroscopic characterization of core/shell QDs. ( a ) TEM images showing typical core/shell QDs with aspect ratios of 0.27, 0.4 and 0.52, and a constant overall radius of 4 nm. Scale bars, 10 nm. Insets are higher resolution images (scale bars, 2 nm) of individual QDs. ( b ) Absorption spectra for the same QDs, indicating a blue shift and a decrease in amplitude of the first excitonic peak associated with the 1 S e −1 S h transition with increasing shell thickness. Spectra are shifted vertically for clarity. ( c ) PL spectra for the same QDs, showing progressive blue shifts with increasing shell size and the emergence of visible emission for the QDs with the thickest shell (shaded spectra). Inset shows a schematic representation of the band structure, indicating the transitions associated with the infrared and visible emission. All infrared spectra are normalized, whereas for the thick-shell structure the visible emission amplitude is multiplied by a factor of 60 for the purpose of comparison. ( d ) Infrared PL traces (core emission) are characterized by microsecond time constants and indicate a progressive increase in single-exciton lifetime (from 0.42 to 1.2 μs, and then 2.6 μs for the plotted traces) for structures with larger shell thicknesses, which is a typical signature of a quasi-type-II regime. ( e ) The PL quantum yield of the infrared band increases with increasing aspect ratio. Full size image Spectroscopic measurements of these QDs conducted as a function of increasing ρ reveal typical signatures of a transition to a quasi-type-II localization regime. As H increases, the band-edge 1S absorption peak shifts to the blue due to increased spatial confinement of the band-edge hole state ( Fig. 3b ) and becomes progressively weaker until it completely vanishes for QDs with the thickest shells. The band-edge photoluminescence (PL) also shifts to higher energy ( Fig. 3c ) and its decay becomes progressively longer ( Fig. 3d ), which is accompanied by an increase in the emission quantum yield (up to 5.5% for ρ =0.62; Fig. 3e ). The apparent reduction in 1S-absorption oscillator strength and increase in PL lifetime are both consistent with expectations for a quasi-type-II system exhibiting progressively increased electron-hole separation. The most striking effect of increasing shell thickness is the development of measureable emission in the visible, which occurs for ρ >~0.45. This new band is observed simultaneously with infrared emission ( Fig. 3c , shaded spectra, and Fig. 4a ). Although initially observed as a broad, weak band consistent with some contribution from emission associated with localized traps within the band gap of the CdSe shell, the emission grows stronger and progressively narrower with shell thickness, while also shifting to lower energy, approaching, yet remaining above, the bulk band gap of CdSe. Simultaneously, we observe a sharp increase in the quantum yield of the visible band ( Fig. 4b ). Together, these characteristics strongly support emission involving an electron in the conduction band-edge state and an unrelaxed (hot) valence band hole residing in the CdSe shell. Normally, because of extremely fast intraband relaxation, hot emission from QDs is only observed in ultrafast spectroscopic measurements; the fact that in these structures it is seen under low-intensity continuous-wave excitation suggests a dramatic slowing of intraband thermalization compared with standard QDs, similar to other heterostructures exhibiting dual-band emission [48] , [49] . 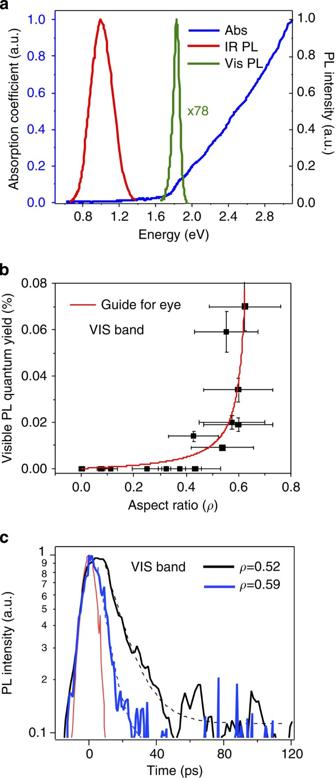Figure 4: Spectral and temporal characteristics of shell-related visible PL. (a) Absorption (blue line) and two-band PL (red and green lines) spectra of a thick-shell PbSe/CdSe QD sample withρ=0.64. (b) Visible PL quantum yields plotted as a function of aspect ratio show a sharp growth of the emission efficiency forρ>0.5, suggesting a significant reduction in the intraband cooling rate for shell-localized holes; horizontal and vertical error bars are defined by, respectively, the QD sample size dispersion (s.d. of aspect ratios based on TEM studies) and the noise level (evaluated in terms of s.d.) of the measurements factoring into the PL quantum yield determination. (c) Dynamics of visible PL originating from the CdSe shell is controlled by relaxation of shell-localized holes. Relaxation time constants for samples withρ=0.52 and 0.59 are 6 ps (blue traces) and 10 ps (black traces), respectively (solid lines are the measurements, dashes are the exponential fits); red line is the measured pump pulse, which defines the width of the instrument response function. All spectroscopic measurements were conducted using low excitation powers for which the average per-dot excitonic occupancy did not exceed 0.1. Figure 4: Spectral and temporal characteristics of shell-related visible PL. ( a ) Absorption (blue line) and two-band PL (red and green lines) spectra of a thick-shell PbSe/CdSe QD sample with ρ =0.64. ( b ) Visible PL quantum yields plotted as a function of aspect ratio show a sharp growth of the emission efficiency for ρ >0.5, suggesting a significant reduction in the intraband cooling rate for shell-localized holes; horizontal and vertical error bars are defined by, respectively, the QD sample size dispersion (s.d. of aspect ratios based on TEM studies) and the noise level (evaluated in terms of s.d.) of the measurements factoring into the PL quantum yield determination. ( c ) Dynamics of visible PL originating from the CdSe shell is controlled by relaxation of shell-localized holes. Relaxation time constants for samples with ρ =0.52 and 0.59 are 6 ps (blue traces) and 10 ps (black traces), respectively (solid lines are the measurements, dashes are the exponential fits); red line is the measured pump pulse, which defines the width of the instrument response function. All spectroscopic measurements were conducted using low excitation powers for which the average per-dot excitonic occupancy did not exceed 0.1. Full size image Using a streak camera we were able to time-resolve shell emission for the samples with the thickest shell ( ρ >0.5), which yielded PL lifetimes of 6–10 ps ( Fig. 4c ). Based on these measurements, we estimate the shell emission quantum yield of 0.03 to 0.05%, if we assume that the radiative time constant of the transition involving the shell-localized hole is close to that of standard CdSe QDs (~20 ns [50] ). This estimation is in line with direct quantum yield measurements, which produced values of 0.01 to 0.07% for samples with ρ >0.5 ( Fig. 4b ). Although both core and shell PL bands involve the same band-edge electron state (inset of Fig. 3c ), their dynamics are dramatically different (compare Figs 3d and 4c ). This implies that the shell emission lifetime is controlled by relaxation of a shell-localized hole and further suggests that the hole residence time in the shell region is at least 6–10 ps. As in these thick-shell structures CM might also contribute to relaxation of shell-localized holes ( Fig. 2a ), the characteristic time of hole cooling via non-CM processes is likely to be even longer than that extracted from the visible PL dynamics. Although being short compared with typical radiative dynamics, the measured relaxation of hot, shell-localized holes is considerably longer than intraband relaxation in core-only PbSe QDs, in which 1P-to-1S relaxation occurs in 0.25–2.6 ps (depending on the QD size) [51] . The relaxation constants at higher, CM-relevant energies are expected to be even shorter due to decreased spacing between electronic states. Thus, the measured hot hole lifetimes of at least 6–10 ps indicate a significant slowing of intraband cooling, which should translate into increased multiexciton yields. Auger recombination lifetimes In these PbSe/CdSe core/shell structures, CM is also expected to benefit from enhanced carrier–carrier Coulomb interactions compared with PbSe QDs of the same overall size. This enhancement is evident from the ρ -dependence of lifetimes of biexciton Auger recombination ( τ 2A ), a Coulombic process in which the energy released during recombination of an electron-hole pair is transferred to a third charge (an electron or a hole). In quasi-type-II structures with more strongly confined holes, Auger recombination is dominated by the hole excitation pathway [49] ( Fig. 5a ), and thus involves scattering processes very similar to those of CM initiated by a hot hole ( Fig. 2a ). Therefore, as was proposed in our earlier work [31] , [39] , [52] , the biexciton Auger lifetimes can be a surrogate for evaluating relative changes in the CM time constant, τ CM , as a function of changes in the QD structure. Indeed, we find that for PbSe/CdSe QDs with large aspect ratios, that is, small core radii (1.42–2.35 nm), the biexciton Auger lifetime is approximately three times shorter than that for standard PbSe QDs of the same total size ( Fig. 5b ). This is consistent with our expectation that Coulomb coupling between the valence-band charges becomes enhanced in thick-shell PbSe/CdSe QD samples, which should also enhance the CM channel involving a hot hole ( Fig. 2a ). 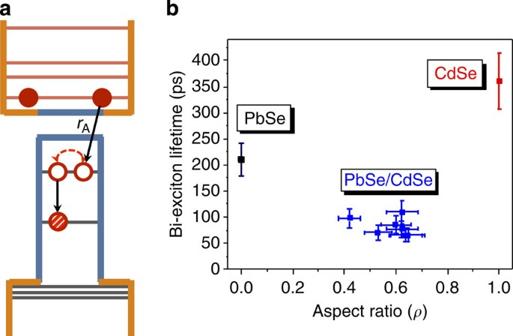Figure 5: Auger decay in core/shell PbSe/CdSe QDs compared with core-only samples. (a) Schematic representation of biexciton Auger decay in a thick-shell PbSe/CdSe QD. In these structures, it is dominated by Coulomb scattering between the two core-localized holes whereby one hole is transferred to the conduction band and the other is excited within the valence band. For the structures with enhanced CM (ρ=0.6–0.7), the excess energy is not sufficiently high to promote the hole above the CdSe valence-band edge. (b) The measured biexciton lifetimes as a function of aspect ratio for the PbSe/CdSe structures with the same overall radius of 4 nm andρfrom 0.42 to 0.64 (blue symbols). The black and red symbols correspond to core-only PbSe and CdSe QDs, respectively; for both samples the QD radius isca. 4 nm, that is, similar to the total radius of the core/shell structures. Theτ2Aconstants measured for the PbSe/CdSe core/shell QDs are considerably shorter compared with those for either core-only PbSe or CdSe QDs, indicating an increase in CM-relevant Coulomb coupling between core-localized charges. Horizontal and vertical error bars are defined by, respectively, the QD samples’ size dispersion (from TEM measurements) and the quality of the exponential fits (least squares method, using a global fit across all fluences) to the measured biexciton dynamics. Figure 5: Auger decay in core/shell PbSe/CdSe QDs compared with core-only samples. ( a ) Schematic representation of biexciton Auger decay in a thick-shell PbSe/CdSe QD. In these structures, it is dominated by Coulomb scattering between the two core-localized holes whereby one hole is transferred to the conduction band and the other is excited within the valence band. For the structures with enhanced CM ( ρ =0.6–0.7), the excess energy is not sufficiently high to promote the hole above the CdSe valence-band edge. ( b ) The measured biexciton lifetimes as a function of aspect ratio for the PbSe/CdSe structures with the same overall radius of 4 nm and ρ from 0.42 to 0.64 (blue symbols). The black and red symbols correspond to core-only PbSe and CdSe QDs, respectively; for both samples the QD radius is ca . 4 nm, that is, similar to the total radius of the core/shell structures. The τ 2A constants measured for the PbSe/CdSe core/shell QDs are considerably shorter compared with those for either core-only PbSe or CdSe QDs, indicating an increase in CM-relevant Coulomb coupling between core-localized charges. Horizontal and vertical error bars are defined by, respectively, the QD samples’ size dispersion (from TEM measurements) and the quality of the exponential fits (least squares method, using a global fit across all fluences) to the measured biexciton dynamics. Full size image CM measurements Experimental measurements indeed indicate a considerable increase in the CM efficiency in PbSe/CdSe heterostructures compared with standard PbSe QDs. In Fig. 6a , we show multiexciton yields (η= q −1, where q is the number of electron-hole pairs generated per absorbed photon) measured using transient PL for PbSe/CdSe core/shell structures (squares) of various aspect ratios but similar band gaps (0.87±0.02 eV), compared with measurements of same- E g core-only PbSe QDs (red line) and nanorods (blue line; interpolated from the data of ref. 34 ); in all measurements the excitation energy is 3.1 eV, which corresponds to ħω / E g of ca . 3.5. For the thinnest-shell sample ( ρ =0.15), the multiexciton yield is only slightly higher than that for the core-only QDs but still lower than that for the nanorods. The value of η increases with ρ , and this growth is especially fast when the aspect ratio exceeds 0.4–0.5. This corresponds to the range of slowed cooling where the core/shell structures exhibit dual infrared and visible emission. For ρ of 0.68, the multiexciton yield reaches the value of 0.75, which is almost four times that in the core-only QDs and twice as large as in the nanorods. 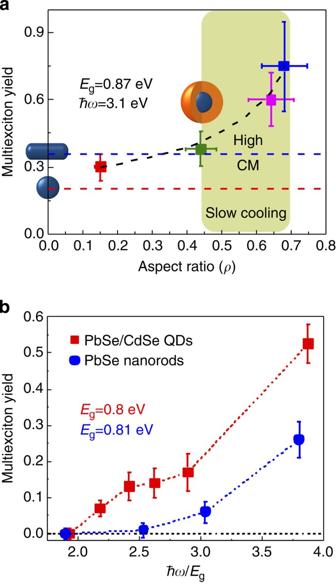Figure 6: CM efficiency for core/shell QDs of varying aspect ratios. (a) Multiexciton yields measured for PbSe/CdSe core/shell structures with progressively increasing shell thicknesses (3.1 eV excitation). The QDs have different total sizes but similar band gaps (~0.87 eV) for proper comparison and are represented by different colour squares on the plot (black dashed line is a guide to the eye). The region where energy conservation is met and, simultaneously, slow cooling is observed (green shading) corresponds to the highest CM yields. The CM yields for PbSe QDs and PbSe nanorods (as interpolated from ref.34) of similar band gaps are shown by red and blue dashed lines, respectively. Horizontal and vertical error bars are defined by, respectively, the QD samples’ size dispersion (from TEM studies) and the quality of the modified Poissonian fits (according to a previously reported method52) to the measured exciton multiplicities plotted as a function of pump fluence. (b) CM threshold measurements for a core/shell sample withEg=0.8 eV (red squares) and PbSe nanorods withEg=0.81 eV (blue circles) using the output of a tunable parametric amplifier, as well as the fundamental-frequency and the second-harmonic outputs of a Ti:sapphire laser (vertical error bars are determined in same way as ina). These data indicate a significant reduction of the CM threshold in the core/shell QDs, approaching the fundamental 2Eglimit. The CM threshold in the nanorods isca. 2.5Eg. Figure 6: CM efficiency for core/shell QDs of varying aspect ratios. ( a ) Multiexciton yields measured for PbSe/CdSe core/shell structures with progressively increasing shell thicknesses (3.1 eV excitation). The QDs have different total sizes but similar band gaps (~0.87 eV) for proper comparison and are represented by different colour squares on the plot (black dashed line is a guide to the eye). The region where energy conservation is met and, simultaneously, slow cooling is observed (green shading) corresponds to the highest CM yields. The CM yields for PbSe QDs and PbSe nanorods (as interpolated from ref. 34 ) of similar band gaps are shown by red and blue dashed lines, respectively. Horizontal and vertical error bars are defined by, respectively, the QD samples’ size dispersion (from TEM studies) and the quality of the modified Poissonian fits (according to a previously reported method [52] ) to the measured exciton multiplicities plotted as a function of pump fluence. ( b ) CM threshold measurements for a core/shell sample with E g =0.8 eV (red squares) and PbSe nanorods with E g =0.81 eV (blue circles) using the output of a tunable parametric amplifier, as well as the fundamental-frequency and the second-harmonic outputs of a Ti:sapphire laser (vertical error bars are determined in same way as in a ). These data indicate a significant reduction of the CM threshold in the core/shell QDs, approaching the fundamental 2 E g limit. The CM threshold in the nanorods is ca . 2.5 E g . Full size image For the considered shell-hole initiated CM pathway, energy conservation is only met within the range of aspect ratios up to a certain critical value ( ρ c ) defined by the condition that the energy released during hole relaxation from the shell- to the core-localized state is greater than or equal to the QD band gap ( Fig. 2a ). Our estimations show that for the QDs with R =4 nm, ρ c is ca . 0.7. This suggest that the range of the optimal aspect ratios where both conditions, slowed cooling and energy conservation, are met corresponds to ρ from ~0.45 to ~0.7 (shown as a shaded area in Fig. 6a ). As we pointed out earlier, a significant asymmetry between the conduction and valence bands of core/shell PbSe/CdSe QDs is expected to lead to a reduction of the CM threshold as compared with that for the core-only QDs or the nanorods. To evaluate the CM threshold, we have measured multiexciton yields as a function of absolute photon energy using excitation with a spectrally tunable optical parametric amplifier. We applied these measurements to PbSe/CdSe QDs and PbSe nanorods with similar band-gap energies of 0.8 and 0.81 eV, respectively ( Fig. 6b ). For ħω =3.1 eV ( ħω / E g is ~3.8), the measured values of η are 0.52 and 0.26 for the core-shell and the nanorod samples, respectively. For both samples, the multiexciton yield gradually decreases with decreasing ħω . For the nanorods, η drops to almost zero at ħω / E g =2.5, suggesting that the CM threshold is close to this value. On the other hand, the core/shell sample shows a non-zero CM efficiency at 1.75 eV ( η is ~7%), which corresponds to ħω / E g of only 2.18. These measurements indicate that in the core/shell QDs, the CM threshold is between 1.94 E g and 2.18 E g , that is, very close to the fundamental 2 E g limit and appreciably lower than in both core-only PbSe QDs and PbSe nanorods. This further implies that using our newly developed infrared-active core/shell nanostructures, high CM yields can be realized at energies well below the high-energy cut-off in the solar spectrum. A considerable slowing down of intraband relaxation in thick-shell samples, which underlies the observed CM enhancement, probably relates to the ρ -dependent interplay between core- versus shell localization of valence-band states. Specifically, our modelling indicates that for ρ >0.4–0.5 the lowest energy hole states (1 S h and 1 P h in Fig. 2a ) still remain mostly core localized, while higher energy states (1 D h , 2 S h and so on in Fig. 2a ) are expelled from the core and become primarily shell localized, which decouples them from the band-edge levels. The coupling between these two types of states is further reduced because of a sizable energetic gap (Δ E cool in Fig. 2a ), which develops between them at large aspect ratios. These peculiar behaviours of valence-band states facilitate accumulation of a long-lived population of shell-localized holes near the CdSe valence-band edge, which explains the development of fairly efficient shell emission and the observed enhancement in CM. Although in the present study we have used PbSe/CdSe QDs, the demonstrated approach to CM engineering through control of intraband cooling and Coulomb interactions is general and can be implemented with other combinations of materials and/or nanostructure geometries. Specifically, we anticipate that a further enhancement in CM should be possible by combining the above approach with other demonstrated means for increasing CM yields such as the use of elongated nanocrystals (nanorods) [34] and/or semiconductors characterized by reduced rates of intraband energy losses (for example, PbTe) [39] . Applied together, these strategies might provide a practical route to designing nanostructures with CM efficiency at or near the ultimate limit as defined by energy conservation. Materials Oleic acid (OA, technical grade 90%), lead(II) oxide (99.999%), cadmium oxide (99.998%) and selenium shot (99.999%) were purchased from Alfa Aesar; 1-octadecene (ODE, technical grade 90%) was purchased from Acros Organics; Tributylphosphine (97%) was purchased from Sigma-Aldrich; Trioctylphosphine (TOP, 97%) was purchased from Strem. QD synthesis PbSe QDs with 3.5–5 nm radii were synthesized from a reported method [47] with modification. A selenium precursor solution (TOPSe, 2 M) was prepared by dissolving 7.896 g selenium shot in 50 ml TOP by stirring for 20 h. Lead(II) oxide (0.892 g) was dissolved in a solution containing 4 ml OA and 16 ml ODE at 120 °C under vacuum in a three-neck round bottom flask, then dried at 120 °C for an additional 30 min. The flask was filled with Ar and heated to 180 °C. A solution prepared from 2 ml selenium precursor and 2 ml tributylphosphine was then rapidly injected into the flask. The reaction was kept at 160 °C for 3–5 min, depending on desired size, and then quenched by cooling to room temperature. The QDs were purified twice by precipitating with ethanol and redispersing in toluene. Core/shell PbSe/CdSe QDs were prepared via a modification of a reported method [47] . Cadmium oxide (1.28 g) was dissolved in a solution containing 10 ml of OA and 10 ml of ODE at 260 °C for 30 min. The solution was then dried under vacuum at 120 °C for 1 h. The purified PbSe QDs were added in toluene solution at room temperature, and then the toluene was removed under vacuum. The cation exchange was performed by heating this solution at 130 °C under Ar, with a total reaction time of ~18 h to reach a 2.5-nm-thick shell. Shell-growth progress was monitored by measuring the infrared PL of aliquots taken periodically during the reaction. Structural characterization Synthesized samples were studied using a JEOL 2010 TEM operating at 200 kV. TEM samples were prepared by drop-casting dilute sample solutions onto carbon-coated copper TEM grids. Spectroscopic measurements Steady-state absorption spectra of colloidal suspensions of PbSe/CdSe core/shell QDs in toluene were obtained using a Perkin-Elmer Lambda 950 ultraviolet–visible-NIR spectrophotometer. Infrared PL spectra were collected using a LN 2 -cooled InSb detector with a grating monochromator, with excitation by an 808-nm diode laser. The excitation was mechanically chopped and the signal was enhanced by a lock-in amplifier. Visible PL spectra were recorded using a Horiba Scientific FluoroMax-4 spectrofluorometer with 3.1 eV excitation. Visible PL quantum yield was determined by performing relative measurements with respect to LDS698 in ethanol (quantum yield 41%). The time-resolved infrared PL measurements were carried out using a Coherent RegA-amplified Ti:sapphire laser operating at 250 kHz (pulse width 200 fs), using either the fundamental (1.55 eV) or the second harmonic (3.1 eV) outputs for excitation. The PL was spectrally analysed using a 20-nm bandwidth monochromator and detected by an NbTiN superconducting single-nanowire single-photon detector (operating at 3.5 K) with an instrument response function width of ~60 ps, which was accounted for in the data analysis [33] . Excitation at 1.55 eV was used to generate PL decay traces for the measurement of single exciton and biexciton Auger lifetimes via single photon counting over long (4 μs) and short (264 ns) time windows, respectively. Multiple measurements with progressively larger excitation densities allowed for the extraction of both absorption cross-sections and biexciton lifetimes. A small, fluence-independent initial relaxation component associated with surface trapping was present in some samples, and it was accounted for in the analysis according to previously reported methods [53] . Excitation at 3.1 eV with very low photon densities (<0.1 exciton per QD per pulse on average) was used to generate PL decay traces for measuring CM efficiencies, which were determined by analysing the signal decay due to Auger recombination of multiple electron-hole pairs following single photon excitation [25] . In the measurements of the CM threshold, in addition to the second harmonic of a fundamental output of a Ti:sapphire laser (3.1 eV), we used the spectrally tunable output of an optical parametric amplifier, which allowed us to cover the range of photon energies from 1.74 to 2.31 eV. All time-resolved data were collected using stirred samples to avoid photocharging effects. The lack of contribution from charged states was confirmed by the consistency of extracted biexciton lifetimes for both 1.55 and 3.1 eV excitations of the same samples. How to cite this article: Cirloganu, C. M. et al. Enhanced carrier multiplication in engineered quasi-type-II quantum dots. Nat. Commun. 5:4148 doi: 10.1038/ncomms5148 (2014).